Structure-based mechanism for Na+/melibiose symport by MelB The bacterial melibiose permease (MelB) belongs to the glycoside–pentoside–hexuronide:cation symporter family, a part of the major facilitator superfamily (MFS). Structural information regarding glycoside–pentoside–hexuronide:cation symporter family transporters and other Na + -coupled permeases within MFS has been lacking, although a wealth of biochemical and biophysical data are available. Here we present the three-dimensional crystal structures of Salmonella typhimurium MelB St in two conformations, representing an outward partially occluded and an outward inactive state of MelB St . MelB adopts a typical MFS fold and contains a previously unidentified cation-binding motif. Three conserved acidic residues form a pyramidal-shaped cation-binding site for Na + , Li + or H + , which is in close proximity to the sugar-binding site. Both cosubstrate-binding sites are mainly contributed by the residues from the amino-terminal domain. These two structures and the functional data presented here provide mechanistic insights into Na + /melibiose symport. We also postulate a structural foundation for the conformational cycling necessary for transport catalysed by MFS permeases in general. Membrane transport proteins from the glycoside–pentoside–hexuronide:cation symporter family [1] , [2] (TC 2.A.2; Supplementary Fig. S1a,b ) are widely found in all life forms, and Escherichia coli melibiose permease (MelB Ec ) is the best-studied representative. However, our understanding of transport mechanisms with these important permeases is limited by lack of high-resolution structures. Salmonella typhimurium MelB (MelB St ) has >85% primary sequence identity with MelB Ec [3] , [4] , and both proteins exhibit ~54% similarity with the human major facilitator superfamily (MFS) domain-containing protein 2A; moreover, the residues essential for transport in MelB are functionally conserved in MFS domain-containing protein 2A [5] . Remarkably different from other MFS transporters [6] , MelB catalyses electrogenic symport of galactosides with Na + , Li + or H + (ref. 7 ); the broad cation selectivity is a prominent feature. Some MelB orthologues selectively couple sugar symport with one or two out of the three cations, but the anomeric configuration of the sugar is important with respect to specific coupling cations [7] . For instance, sugars in the α-configuration (melibiose and raffinose) utilize all three cations, but β-anomers of galactopyranosides couple only to Na + and Li + (ref. 8 ). MelB St shares similarity with regard to cation-coupling specificity and other transport features with the well-studied MelB Ec [4] , [7] , [9] , [10] , [11] , [12] . All three coupling cations compete for a single binding site with a protein/sugar/cation stoichiometry of unity [4] , [13] , [14] . Electrogenic sugar symport is driven by Δ H+, Na+ or Li+ , depending on the coupling cation [4] . Thermodynamically, MelB transduces the free energy from the downhill translocation of a cation to drive translocation of sugar against a concentration gradient and vice versa [4] , [12] . Here we present three-dimensional X-ray crystal structures of MelB St in two distinct conformations, refined to 3.35 Å. The structure is in general agreement with the predicted model of MelB [15] . Notably, most MFS members are either H + symporters or uniporters. Among the members with solved structures [16] , [17] , [18] , [19] , [20] , [21] , [22] , [23] , MelB St is the sole member that utilizes Na + primarily as a coupling cation for symport and uses a previously uncharacterized coupling mechanism. Functional characterization Purified MelB St is monodisperse, stable ( Supplementary Fig. S2a,b ) and binds melibiose, 2′-(N-dansyl)aminoalkyl-1-thio-β- D -galactopyranoside (D 2 G) or methyl-β- D -thiogalactoside, but has no affinity for sugars without a galactopyranosyl moiety ( Fig. 1a ). A single sugar-binding site was determined by isothermal titration calorimetry (ITC; Fig. 1b,c ). Melibiose binding is exothermic with a K d of ~1 mM in the presence of Na + or Li + , which is consistent with previous results [4] . Furthermore, sugar binding is driven energetically by a small favourable enthalpy change (Δ H ) and a bigger increase in entropy (TΔS). 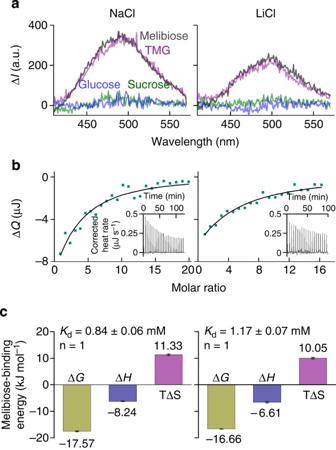Figure 1: Functional characterization. Purified MelBStcontaining 100 mM NaCl or LiCl were subjected to D2G FRET and ITC measurements. (a) D2G FRET measurement. With an excitation wavelength of 290, emission spectra were collected between 415 and 575 nm. Difference spectra (ΔI) were calculated before and after addition of a given sugar (50 mM). Grey curves, melibiose; purple curves, methyl-β-D-thiogalactoside (TMG); green curves, sucrose; blue curves, glucose. (b) ITC measurement. Melibiose titration thermograms (insets) were recorded at 25 °C. Cumulative heat change (ΔQ) is plotted as a function of the molar ratio of melibiose/MelBSt, and fitted with the one-site independent binding model. (c) Melibiose-binding energetics. Enthalpy change (ΔH) and the association constant (Ka) were measured directly; dissociation constantKd=1/Ka; free-energy change ΔG=−RT lnKa; entropy change ΔTS=ΔH−ΔG;n, stoichiometry. Error bar, s.d.,n=2. Figure 1: Functional characterization. Purified MelB St containing 100 mM NaCl or LiCl were subjected to D 2 G FRET and ITC measurements. ( a ) D 2 G FRET measurement. With an excitation wavelength of 290, emission spectra were collected between 415 and 575 nm. Difference spectra (Δ I ) were calculated before and after addition of a given sugar (50 mM). Grey curves, melibiose; purple curves, methyl-β- D -thiogalactoside (TMG); green curves, sucrose; blue curves, glucose. ( b ) ITC measurement. Melibiose titration thermograms (insets) were recorded at 25 °C. Cumulative heat change (Δ Q ) is plotted as a function of the molar ratio of melibiose/MelB St , and fitted with the one-site independent binding model. ( c ) Melibiose-binding energetics. Enthalpy change (Δ H ) and the association constant ( K a ) were measured directly; dissociation constant K d =1/ K a ; free-energy change Δ G =−RT ln K a ; entropy change ΔTS=Δ H −Δ G ; n , stoichiometry. Error bar, s.d., n =2. Full size image Overall fold of MelB St The structure of MelB St was solved by molecular replacement and refined to a resolution of 3.35 Å ( Table 1 ). The asymmetric unit contains four molecules (Mol-ABCD; Supplementary Fig. S3a,b ) with twinning and pseudotranslation symmetries. Surprisingly, twinned Mol-B and Mol-D have a conformation different from Mol-A and Mol-C ( Fig. 2 and Supplementary Fig. S4a,b ). We describe only Mol-A and Mol-B here as representative structures. Table 1 Data collection and refinement statistics (molecular replacement). 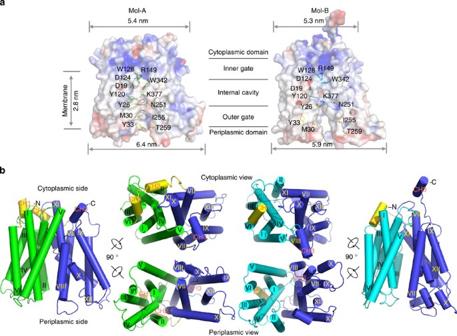Figure 2: Crystal structures of MelBStin two outward conformations. (a) Surface electropotential maps with side chains forming the outer gate and the internal cavity shown in yellow and green (Mol-A), respectively, or cyan (Mol-B) sticks. (b) Overall structure of MelBSt. The N-terminal domains of Mol-A or Mol-B are shown in green and cyan, respectively, and the central loops are shown in yellow. The helices are labelled with Roman numerals. CH1–3 denote the helices in the cytoplasmic loops and the C-terminal tail. All figures showing MelB structures were prepared by Cα1–430superposition of Mol-B on Mol-A. Full size table Figure 2: Crystal structures of MelB St in two outward conformations. ( a ) Surface electropotential maps with side chains forming the outer gate and the internal cavity shown in yellow and green (Mol-A), respectively, or cyan (Mol-B) sticks. ( b ) Overall structure of MelB St . The N-terminal domains of Mol-A or Mol-B are shown in green and cyan, respectively, and the central loops are shown in yellow. The helices are labelled with Roman numerals. CH1–3 denote the helices in the cytoplasmic loops and the C-terminal tail. All figures showing MelB structures were prepared by Cα 1–430 superposition of Mol-B on Mol-A. Full size image As predicted [15] , MelB St adopts a typical MFS fold, organized in amino- and carboxy-terminal six-transmembrane α-helix bundles (Fig. 2), with a connecting cytoplasmic central loop containing two short helices (CH1 and CH2), and the cytoplasmic C-terminal tail with another short α-helix (CH3). Both the N and C termini are on the cytoplasmic side of the membrane and the overall shape is consistent with the electron-microscopic map of MelB Ec [24] . The N- and C-terminal domains are related by a pseudo two-fold symmetry axis perpendicular to the membrane plane and separated from each other by an internal cavity facing the periplasm. Within each domain, there is a two-fold inverted pseudosymmetry between helices I–III and IV–VI, as well as between VII–IX and X–XII, forming repeats A–D (Supplementary Fig. S4c). Similar to other MFS members [16] , [18] , [25] , MelB may have evolved from triple-helix repeats with a similar genetic origin. Most MelB St helices are irregular with kink(s) and tilts ( Fig. 2b and Supplementary Figs S3 and S4 ). Two to three broken helices are observed in both molecules: helices IV, X and XI in Mol-A and helices II, VII and X in Mol-B. Mol-A exhibits a periplasmic-facing conformation with a partially occluded internal cavity due to the interactions between helices I and VII in the N- and C-terminal domains, respectively. This structure is described as an outward partially occluded conformation ( Figs 2a and 5c). The cavity is closed on the cytoplasmic side by interdomain contacts between inner helices IV/X, V/VIII and II/XI; solvent is accessible from the periplasmic side. Mol-B has a partial outward opening compared with fully opened FucP [20] , and is described as a partial outward conformation ( Figs 2a and 5c). The root mean squared deviation between Mol-A and Mol-B is 2.7 Å, and the major differences are found in the first two helices of each repeat ( Supplementary Fig. S4c ), indicating that the inner helices move relatively independently between the two conformations. Viewed from the periplasmic side, the internal cavity in Mol-A has an asymmetric charge distribution ( Fig. 3a ). Except for Lys377 in the C-terminal domain, all other charged residues, including Asp residues (19, 55, 59 and 124), Lys18 and Arg residues (52 and 149), are in the N-terminal domain. The calculated omit maps do not reveal interpretable densities for either bound sugar or cation. 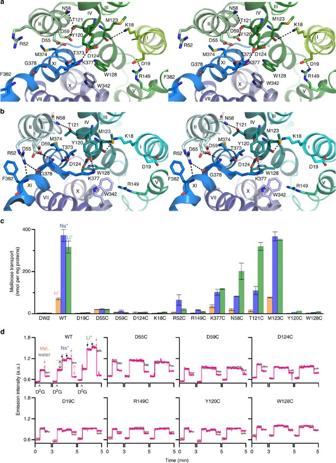Figure 3: Cosubstrate-binding sites. (a) Wall-eyed stereo view from the periplasmic side of the internal cavity in Mol-A with the N- and C-halves in green and blue, respectively. (b) Identical view of Mol-B with N- and C-halves in cyan and blue, respectively. (c) Steady-state levels of [3H]melibiose accumulation by intact cells at 10 min presented as histograms. DW2, cells without MelB. Error bar, s.e.m.;n=2 for all mutants with a single-site mutation andn=10 for the WT and DW2. (d) Trp→D2G FRET with RSO vesicles. The emission signals were collected at wavelength of 490 nm after being excited at wavelength of 290 nm. ⁁, adding 10 μM D2G; pink arrows ↓, adding 120 mM melibiose; grey arrows ↓, adding water; black arrows ↓, adding 20 mM or 50 mM Na+or Li+. Black double-headed arrows ↔, Na+or Li+stimulation; pink double-headed arrows ↔, melibiose displacement of D2G. Figure 3: Cosubstrate-binding sites. ( a ) Wall-eyed stereo view from the periplasmic side of the internal cavity in Mol-A with the N- and C-halves in green and blue, respectively. ( b ) Identical view of Mol-B with N- and C-halves in cyan and blue, respectively. ( c ) Steady-state levels of [ 3 H]melibiose accumulation by intact cells at 10 min presented as histograms. DW2, cells without MelB. Error bar, s.e.m. ; n =2 for all mutants with a single-site mutation and n =10 for the WT and DW2. ( d ) Trp→D 2 G FRET with RSO vesicles. The emission signals were collected at wavelength of 490 nm after being excited at wavelength of 290 nm. ⁁, adding 10 μM D 2 G; pink arrows ↓, adding 120 mM melibiose; grey arrows ↓, adding water; black arrows ↓, adding 20 mM or 50 mM Na + or Li + . Black double-headed arrows ↔, Na + or Li + stimulation; pink double-headed arrows ↔, melibiose displacement of D 2 G. Full size image The cation-binding site A cluster of Asp residues at positions 55 and 59 (helix II), and 124 (helix IV), forms a pyramidal-shaped pocket in Mol-A ( Fig. 3a and Supplementary Fig. S5a ). In close proximity, there are Tyr120, Thr121 (helix IV) and Thr373 (XI). Together these residues could form the trigonal bipyramid geometry required for a metal-binding site [26] , [27] . Thr121 forms H-bonds with Asn58 and Asp59, stabilizing the interaction between helices II/IV, and Lys377 H-bonds with Tyr120 separating the negatively charged pocket from the central water-filled cavity ( Fig. 3a ). Asp124 is buried between Tyr120 and Trp128. Asp59 is buried in a hydrophobic environment ( Supplementary Fig. S5c ). Remarkably, Cys replacement at position 55, 59, 124, 58, or 121 differentially alters cation selectivity. Thus, the D55C mutant in MelB St retains only a low level of H + -coupled melibiose binding and active transport ( Fig. 3c,d and Supplementary Fig. S6a ), but Na + or Li + does not stimulate either binding or transport. The D59C and D124C mutants bind ligand with reduced affinity ( Fig. 3d ), but do not catalyse active melibiose transport ( Fig. 3c and Supplementary Fig. S6a ). Reduced rates of melibiose efflux and exchange are observed with mutant D59C, but mutant D124C does not exhibit exchange activity. In contrast to wild type (WT), melibiose binding, efflux and exchange in the D59C mutant are not stimulated by Na + or Li + nor is efflux inhibited at acidic pH ( Fig. 4 ); thus, the D59C mutant behaves similar to a sugar uniporter. None of these mutations has an adverse effect on protein expression ( Supplementary Fig. S6b ). Furthermore, both the N58C and T121C mutations selectively inhibit H + - and Na + -coupled activity, with little effect on Li + -coupled melibiose transport ( Fig. 3c and Supplementary Fig. S6a ). Combined with the observed geometry and functional data presented here and elsewhere [7] , [28] , [29] , [30] , we propose that the cation-binding site selectively coordinates Na + , Li + or H 3 O + through a dynamic change in size and shape [27] dictated by the orientation of Asp55, Asp59 and Asp124. This supports the conclusion that all coupling cations in MelB compete for a single binding site [4] , [13] , [14] . It is apparent that each Asp residue at these positions has a specific role in cation binding and coupling. All three Asp residues are required for Na + or Li + binding, and Asp59 is essential for H + binding. Asp59 is buried in a hydrophobic environment ( Supplementary Fig. S5c ); based on the PROPKA prediction [31] , it has a largely elevated pKa of 9.0. We propose that Mol-A is in a protonated state. As the cation-binding site binds H + , Na + or Li + mutually exclusively [4] , [13] , [14] , a bound Na + is not expected in this configuration. 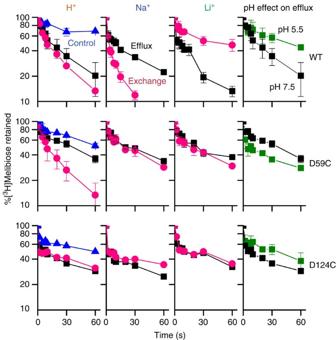Figure 4: Melibiose efflux and exchange. RSO membrane vesicles (28 mg ml−1) containing MelBStwere tested for outwardly directed flow of [3H]melibiose in the absence (efflux, squares) or presence (exchange, red circles) of equimolar concentration of unlabelled melibiose. The same experiment was performed in the presence of 20 mM NaCl or LiCl. 2-(4′-maleimidylanilino)naphthalene-6-sulphonic acid-treated vesicles were used for the negative control (blue triangles). Acidic pH effect on melibiose efflux was tested by decreasing the dilution buffer pH to 5.5 (green squares). Error bar, s.e.m.,n=2. Figure 4: Melibiose efflux and exchange. RSO membrane vesicles (28 mg ml −1 ) containing MelB St were tested for outwardly directed flow of [ 3 H]melibiose in the absence (efflux, squares) or presence (exchange, red circles) of equimolar concentration of unlabelled melibiose. The same experiment was performed in the presence of 20 mM NaCl or LiCl. 2-(4′-maleimidylanilino)naphthalene-6-sulphonic acid-treated vesicles were used for the negative control (blue triangles). Acidic pH effect on melibiose efflux was tested by decreasing the dilution buffer pH to 5.5 (green squares). Error bar, s.e.m., n =2. Full size image In Mol-B, the pyramidal-shaped cation-binding site is deformed. Displacement of the helix XI kink between helices II and IV places Asp55 and Asp59 in a different environment ( Fig. 3b and Supplementary Fig. S5d ), distorting the pyramidal arrangement. The deformation of the cation-binding site is probably necessary to release the bound Na + . This conformational change, which is involved in rearrangement of the helices, is expected to contribute to the rate-limiting step of transport [4] , [9] , [32] . In this state, Arg52 holds helix XI by H-bonding with backbone atom of Gly378, indicating a primary structural role. Furthermore, Asp55 also stabilizes packing between helices II and XI. The known crystal structures of other Na + -coupled symporters [26] , [33] , [34] have a relatively low-affinity Na + -binding motif, where four to six partial charges coordinate Na + . In contrast, MelB utilizes three Asp residues representing a unique, higher-affinity Na + -binding motif [4] , [29] . The sugar-binding site The sugar specificity of MelB St is highly selective for di- or trisaccharides containing a D -galactopyranosyl moiety or the monosaccharide D -galactose, as in MelB Ec [8] or LacY [35] , [36] , [37] . In close proximity to the cation-binding site, a water-filled cavity is observed between residues Asp19 (helix I), Arg149 (helix V), Tyr120, Asp124 and Trp128 (helix IV), as well as Lys377 (helix XI; Fig. 3a ). Asp19 and Arg149 form a salt bridge on one side of the cavity; Tyr120 and Lys377 are H-bonded on the other side. Cys replacement at each of these positions abolishes or markedly decreases binding, as measured by Trp→D 2 G fluorescence resonance energy transfer (FRET), and melibiose transport ( Fig. 3c,d , and Supplementary Figs S6 and S7 ), although mutant K377C retains 30–40% of WT symport activity with each cation ( Fig. 3c and Supplementary Fig. S6a ). In MelB Ec , single-Cys mutation of Asp19 selectively abolishes sugar binding with little effect on Na + binding [30] , mutant W128F has decreased affinity for 4-nitrophenyl-α- D -galactopyranoside [38] , and mutants Y120F and D124E exhibit decreased sugar- and Na + -binding affinities [39] . Therefore, these charged or polar side chains, particularly Asp19 and Arg149, play critical roles in sugar selectivity and affinity, and the aromatic residues Trp128 and Tyr120 may contribute to affinity by CH/π-interactions with the pyranosyl ring of the sugar [40] , [41] . Clearly, a crystal structure with bound sugar is required to determine the sugar-binding coordinates precisely. In Mol-B, the salt bridge between Asp19 and Arg149 is broken, and Trp128 is also displaced from the cavity, suggesting deformation of the sugar-binding site ( Fig. 3b ). It is noteworthy that the cation-binding site is also collapsed in this conformation; hence, the Mol-B probably represents an inactive state of MelB St . It is interesting that both LacY and MelB have similar sugar specificity and location of the sugar-recognition sites [35] ; however, their cation-binding sites are related by a pseudo two-fold symmetry axis perpendicular to the membrane plane. The location of the Na + -binding site in MelB is away from Arg149, which is involved in sugar binding, thereby allowing the presence of a strongly negatively charged metal-binding site without a negative influence on sugar binding. Positive cooperative binding between the cosubstrates is well established in MelB [4] , [38] , [39] , [42] . Helix IV, in the middle of the N-terminal domain, physically connects both cosubstrate sites. In addition to Tyr120 and Asp124, Lys18 ( Fig. 3c and Supplementary Fig. S6 ) H-bonds with the backbone atom of Met123 ( Fig. 3a,b ), which links helices I–IV, underscoring the crucial role of helix IV in cooperative binding and transport. On the basis of the structures, we anticipate that Na + binding leads to movement of helix IV, which recruits Asp124, optimizing the pyramidal shape of the cavity with Asp55 and Asp59, and aligning Tyr120 and Trp128 for aromatic stacking with the sugar, thereby increasing affinity. It is well documented that sugar affinity is increased by more than threefold in the presence of Na + or Li + (refs 4 , 13 , 29 , 30 , 43 ), and Asp124 is required for completion for the Na + -binding site [30] . Ionic locks and conformational cycling Both conformers are present in the same crystal, indicating that MelB St has multiple conformations. Available crystal structures show MFS permeases in inward or outward conformations with occluded or partial-to-fully open cavities ( Fig. 5 ), implying that an individual transporter may favour few conformers within a conformational cluster depending on the lowest free-energy state. The energy barrier for altering conformational equilibrium between inward and outward clusters may be the formation of an occluded intermediate state. Here we show that extramembrane electrostatic interactions play a crucial role in this regard. 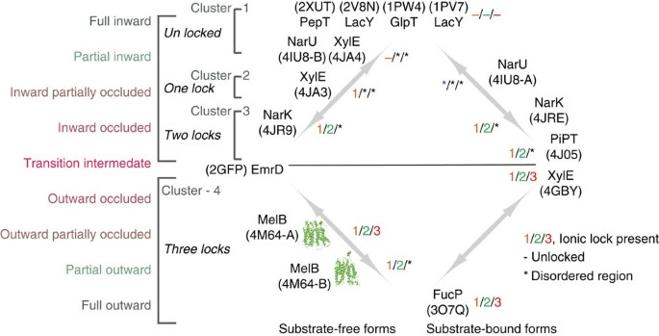Figure 5: Clusters of MFS permeases in different conformations. Structures were categorized into clusters according to their conformational state. *, Disordered region in structure; −, at an unlocked state; 1/2/3, the presence of lock-1, lock-2 or lock-3. PDB ID is shown for each structure. Figure 5: Clusters of MFS permeases in different conformations. Structures were categorized into clusters according to their conformational state. *, Disordered region in structure; −, at an unlocked state; 1/2/3, the presence of lock-1, lock-2 or lock-3. PDB ID is shown for each structure. Full size image Both inside-closed structures of MelB St exhibit multiple hydrophobic interactions (hydrophobic patches) on the cytoplasmic side of the transmembrane helices sealing the cavity between N- and C-domains ( Fig. 6a , left). This sealed dynamic domain is also stabilized by interdomain electrostatic interactions, designated as ionic locks, involving three Arg residues: Arg295 (cytoplasmic end of helix IX), Arg141 (cytoplasmic end of the helix V) and Arg363 (flexible loop 10–11 ; Fig. 6a,b ). At the first ionic lock (L-1), Arg295 forms multiple H-bonds with Gln143 (helix V) and Pro287 (helix VIII) to hold helix V close to the C-terminal domain. At L-2, Arg141 forms four H-bonded ion pairs with Asp351 and Asp354 (helix X), stabilizing helix X. At L-3, Arg363 (loop 10–11 ) forms one ion pair and two H-bonding interactions with the backbone atoms of Val204, Asp208 (N-terminal side of central loop 6–7 ) and Gly74 (loop 2–3 ), holding the N-terminal domain in an outward-facing conformation. It is likely to be that by stabilizing helix X, ionic locks L-1 and L-2 facilitate interaction of Arg363 with its partners. Replacing Arg363, Arg141 or Arg295 individually with Cys yields conformationally compromised mutants that fail to transport but retain affinity for both cosubstrates ( Fig. 6c,d and Table 2 ). As indicated from a thread model of MelB St at an inward-facing conformation ( Fig. 6a , right), all three cytoplasmic interdomain locks are at an unlocked state, as the residues involved in these electrostatic interactions are 20 Å far apart. Therefore, these three ionic locks play important role in facilitating the formation of outward-facing conformation. On the periplasmic side, Asp35 (helix I) organizes L-4 ( Fig. 6a,b ) by forming a salt bridge and an H-bond with Arg175 (helix VI) and stabilizes the outward-facing conformation. 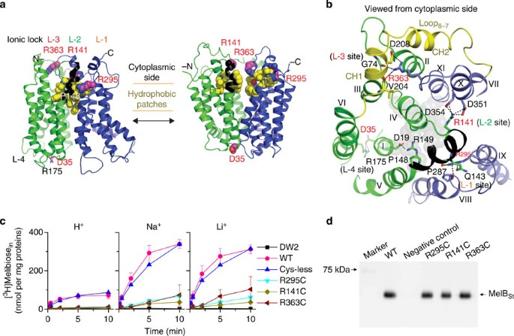Figure 6: Ionic locks and conformational cycling. N- and C-terminal domains are shown in green and blue, respectively, and hydrophobic patches are in yellow. Arg141–Arg149 stretch is coloured as black. ‘L’ denotes positions of ionic locks. (a) Left, outward partially occluded conformation (Mol-A); right, threading model for inward conformation. (b) Residues forming ionic locks are shown in sticks connected by broken lines. Grey spheres represent the residues involved in sugar binding. (c) Cys mutant of Arg residue at position 295, 141 or 363. IntactE. coliDW2 cells containing WT MelBStor a given mutant were assayed for [3H]melibiose transport (0.4 mM, 10 mCi mmol−1) in the absence or presence of 20 mM NaCl or LiCl. Intracellular melibiose expressed as nmol mg−1of total proteins is plotted as a function of time. Each single-site mutation is in the WT background. Error bar, s.e.m.,n=2 for the mutants andn=3 for the WT. (d) Western blotting. Twenty-five micrograms of RSO vesicles was loaded on each well and detected by anti-His-tag antibody. Figure 6: Ionic locks and conformational cycling. N- and C-terminal domains are shown in green and blue, respectively, and hydrophobic patches are in yellow. Arg141–Arg149 stretch is coloured as black. ‘L’ denotes positions of ionic locks. ( a ) Left, outward partially occluded conformation (Mol-A); right, threading model for inward conformation. ( b ) Residues forming ionic locks are shown in sticks connected by broken lines. Grey spheres represent the residues involved in sugar binding. ( c ) Cys mutant of Arg residue at position 295, 141 or 363. Intact E. coli DW2 cells containing WT MelB St or a given mutant were assayed for [ 3 H]melibiose transport (0.4 mM, 10 mCi mmol −1 ) in the absence or presence of 20 mM NaCl or LiCl. Intracellular melibiose expressed as nmol mg −1 of total proteins is plotted as a function of time. Each single-site mutation is in the WT background. Error bar, s.e.m., n =2 for the mutants and n =3 for the WT. ( d ) Western blotting. Twenty-five micrograms of RSO vesicles was loaded on each well and detected by anti-His-tag antibody. Full size image Table 2 Affinity for melibiose and Na + . Full size table Similar ionic lock interactions are present in other MFS structures ( Fig. 5 and Supplementary Fig. S8 ). From top to bottom in the Fig. 5 , conformations are depicted from the full-inward to the full-outward states [17] , [18] , [20] , [21] , [22] , [23] , [44] , [45] , [46] . None of the predicted locks L-1, L-2 and L-3 exists in cluster-1, which includes the full and partially inward states. L-1 is formed in cluster-2, the inward partially occluded state. When the conformation reaches a more occluded state (cluster-3), both L-1 and L-2 are observed. L-3 is not observed in any of the inward conformers, but exists in most outward structures (cluster-4). Thus, formation of an occluded state probably requires L-1 and L-2, and the outward state requires all three ionic locks. Reverse order of lock formation is expected for the conformational changes to proceed in the opposite direction. The formation and deformation of these ionic interactions are the structural foundation for the function-required conformational switching between inward and outward conformers. What triggers the locking/unlocking processes? In MelB, the salt bridge between Arg149 and Asp19 is involved in sugar binding. It is noteworthy that a short cytoplasmic stretch of helix V (Arg141–Arg149) links the sugar-binding site with two ionic locks (L-1 and L-2; Fig. 6a,b ) and also contains two other conformationally important residues, Glu142 (ref. 42 ) and Pro148 (ref. 47 ). We propose that sugar binding promotes a dynamic state of the cytoplasmic stretch of helix V ( Fig. 6a,b ) and triggers locking/unlocking processes associated with a cascade of structural rearrangements for reorientation of the sugar-binding pocket. We previously proposed a sequential binding kinetic model to explain reversible cation/melibiose symport in MelB based on an alternating-access mechanism ( Fig. 7 ) [9] , [12] , [42] . The structural and functional studies discussed here allow integration of the conformational states with kinetic steps in the proposed model for explaining melibiose/Na + symport reactions. Although melibiose/Na + efflux is explained for experimental simplicity [4] , influx is the reverse reaction starting from the intermediate [6] ( Fig. 7 ) and proceeds via the red arrows around the circle; active melibiose transport driven by Δ H+, Na+ or Li+ is likely to occur in similar fashion. The polarity of transport is controlled by the direction of the net free energy stored in the form of either the sugar gradient or the electrochemical gradient of Na + , Li + or H + , and the transport process is reversible. 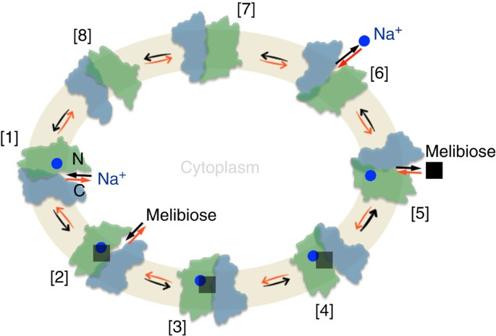Figure 7: Scheme for Na+/melibiose symport. [1–8], Kinetic steps in the overall transport cycle. The green colour-filled cycle represents the cell inner membrane. Na+, blue circles; melibiose, black squares. N, the N-terminal domain in green colour; C, the C-terminal domain in blue colour. Melibiose influx down a sugar concentration gradient starts at step [6] and proceeds via the red arrows around the circle, and melibiose efflux down a sugar concentration gradient starts at [1] and proceeds via the black arrows around the circle. Active transport of melibiose against a concentration gradient proceeds from step [6] via the red arrows as the melibiose influx. Figure 7: Scheme for Na + /melibiose symport. [1–8], Kinetic steps in the overall transport cycle. The green colour-filled cycle represents the cell inner membrane. Na + , blue circles; melibiose, black squares. N, the N-terminal domain in green colour; C, the C-terminal domain in blue colour. Melibiose influx down a sugar concentration gradient starts at step [6] and proceeds via the red arrows around the circle, and melibiose efflux down a sugar concentration gradient starts at [1] and proceeds via the black arrows around the circle. Active transport of melibiose against a concentration gradient proceeds from step [6] via the red arrows as the melibiose influx. Full size image This simplified scheme for melibiose efflux involves eight states ( Fig. 7 , black arrows): [1] inward Na + -bound state. Binding of a Na + to the cation-binding site induces helix IV movement with an increase in sugar affinity. [2] Inward Na + - and melibiose-bound state. Sugar binding from the cytoplasm initiates the locking process ( Fig. 6a,b ). [3] Occluded Na + - and melibiose-bound state. Closure of the cytoplasmic cavity by the hydrophobic patch is locked by L-1 and L-2. [4] Outward Na + - and melibiose-bound state. Interactions at L-3 and L-4 facilitate a conformational transition from the occluded to an outward state. [5] Outward melibiose-released state. Bound melibiose is released to the periplasmic side from the open outer gate. The crystal structures of MelB St suggest that the cation exits via the internal cavity that contains the sugar-binding site and that a bound sugar should restrain the dynamics of the bound cation; therefore, release of sugar is a prerequisite for releasing Na + . The structural basis for the ordered release is supported by kinetic studies [4] , [11] and the behaviour of mutant G117R [9] , which catalyses melibiose exchange but no reaction involving net Na + transport, that is, involving only steps [1] ⇔ [5]. [6] Outward Na + -released state. Deformation of the cation-binding site facilitates Na + release as suggested by the Mol-B structure ( Fig. 3b ). [7] Occluded-empty state. Formation of the unloaded intermediate state occluded on both sides. [8] Inward-empty state. Once the cavity is open to the cytoplasm, the next transport cycle begins. Melibiose efflux involves the whole cycle with one sugar and one charge moving across the membrane. In contrast, melibiose exchange involves only states [1–5] . Interestingly, it appears that the kinetic model is similar for different MFS permeases regardless of the coupling cation [35] , [48] , [49] . In the solely H + -coupled LacY [50] , [51] , [52] , [53] , it is well established that at physiological pH, LacY is protonated [52] . Sugar binds only to protonated LacY [50] , [53] and dissociates before the release of H + during symport [50] . The inward-facing crystal structures of LacY [16] , [17] indicate that the sugar-binding site is coupled to the H + -binding site through an electrostatic network; as a result, the affinity for the sugar binding is optimized in a protonated state. A similar coupling phenomenon is observed in MelB. The comparison of the structures of Mol-A and Mol-B reveals that a protonated cation-binding site is coupled with a properly formed sugar-binding pocket, and the deformation of the cation-binding site induces deformation of the sugar-binding site. In LacY, the H + may involve in a single side chain (for example, Glu325) [16] , [17] , [35] , [54] ; in MelB, the H + may be bound in different forms, a protonated side chain (for example, Asp59) or as H 3 O + that is shared by Asp55, Asp59 and Asp124 in the metal-binding cavity. Possibly, these two protonation forms represent different states of bound H + in MelB. What is the effect of Na + or Li + on MelB? In general, binding of Na + or Li + requires four to six coordination numbers from two to three helices, and the small ionic radius of Na + and Li + require the coordination ligands in closer distance. Thus, metal binding should induce a relatively large change in movement of helices. On the basis of the structures of MelB St , it is anticipated that Na + binding recruits Asp124 to complete Na + binding, resulting in movement of helix IV with Tyr120 and Trp128 for aromatic stacking with the bound sugar. It is well known that sugar affinity is largely increased by aromatic stacking in LacY [40] . According to this notion, Na + and Li + are more effective ‘activators’ than H + . This structural interpretation is consistent with the previous conclusion derived from functional studies of MelB Ec [30] , [32] , [38] . Therefore, it is likely to be that an essential aspect of coupling is that binding of the cation activates the substrate-binding site, a property that is conserved in both MelB and LacY. What prevents cation leakage in MelB? The opening and closing of the cytoplasmic side to form the substrate exit pathway involves dynamics of cytoplasmic helix V in MelB ( Fig. 6a,b ), which is initiated only by sugar binding. In the absence of sugar, ‘the leader’, MelB/Na + complexes should preferentially populate outward conformations. This structural arrangement can prevent bound Na + from futile cycling and also offers an explanation for how the extramembrane ionic locks, as ‘the follower’, respond to the primary effect of sugar binding in the middle of the molecule. Large-scale protein production Full-length MelB St encoded by plasmid pK95 ΔAH/MelB St /CHis 10 (refs 4 , 55 ) with Leu5→Met and a His 10 tag at the C terminus (namely the WT) was expressed in E. coli DW2 strain ( mel A + , Δ mel B and Δ lac ZY) [55] . In a 10-l fermenter, cells were grown in Luria–Bertani (LB) broth supplemented with 50 mM KP i (pH 7.0), 45 mM (NH 4 )H 2 PO 4 , 0.5% glycerol and 100 mg l −1 ampicillin at 30 °C until they approached stationary phase at A 600 of ~3.3. Cells with constitutively overexpressed MelB St were then harvested, resuspended in 20 mM Tris–HCl (pH 7.5), 200 mM NaCl and 10% glycerol, broken with an EmulsiFlex instrument and centrifuged at 20,000 g for 15 min to remove unbroken cells [56] . Membranes were harvested from the supernatant by ultracentrifugation at 144,651 g for 3 h in a Beckman rotor, type 45 Ti. The pellets were resuspended in the same buffer, frozen in liquid N 2 and stored at −80 °C. The protein concentration of the membrane samples was assayed using Micro BCA Protein Assay Kit (Pierce). Protein purification Membranes (14 mg ml −1 ) were extracted with 1.5% n-undecyl-β- D -maltoside (UDM) followed by ultracentrifugation at 265,000 g for 30 min. Purification was performed by cobalt-affinity chromatography (TALON resins). The column was pre-equilibrated with 50 mM NaP i (pH 7.6), 200 mM NaCl, 10% glycerol, 0.035% UDM, 5 mM imidazole. After loading and washing the column with 35 mM imidazole buffer, MelB St was eluted with buffer containing 200 mM imidazole, concentrated with VIVASPIN 20 (50 kDa cutoff value), dialysed twice against 1 litre of 20 mM Tris–HCl (pH 7.5), 100 mM NaCl, 10% glycerol, 0.035% UDM, further concentrated to >20 mg ml −1 , and finally ultracentrifuged at >360,000 g for 45 min. The protein was flash-frozen in liquid nitrogen and stored at −80 °C. From a 10-l culture, highly purified MelB St at 30–40 mg was obtained routinely. Isothermal titration calorimetry ITC measurements were performed in a nano isothermal titration calorimeter (TA Instruments). The purified MelB St in the dialysis buffer was injected into the ITC sample cell and 6 mM melibiose dissolved in the same dialysis buffer was titrated incrementally into the protein sample, and the heat rate was recorded at 25 °C. Melibiose binding was also measured in the presence of 100 mM LiCl. The cumulative heat change (Δ Q ) was plotted against the molar ratio of melibiose to MelB St and fitted with the one-site independent binding model (NanoAnalyse software). Protein expression for functional studies E. coli DW2 cells containing a given plasmid were grown in LB broth with 100 mg l −1 of ampicillin at 37 °C. The overnight cultures were diluted by 5% to LB broth supplemented with 0.5% glycerol and 100 mg l −1 of ampicillin, and the constitutive overexpression was obtained by shaking at 30 °C for another 5 h. Preparation of right-side-out membrane vesicles RSO membrane vesicles were prepared from E. coli DW2 cells by osmotic lysis [4] , [57] , [58] . Cells were incubated with 50 μg ml −1 lysozyme in the presence of 10 mM EDTA (pH 7.5), 5 mM dithiothreitol (DTT) and 30% (w/v) sucrose for 45 min; the yielded spheroplasts were harvested by centrifugation at 14,000 g for 40 min at 4 °C and suspended with 20-ml cocktail containing 100 mM KP i (pH 7.5), 20 mM MgSO 4 , 30% sucrose, 5 mM DTT, 1 mg ml −1 deoxyribonuclease and 1 mg ml −1 ribonuclease. The resuspended spheroplasts were lysed by rapid dilution into 1-litre 50 mM KP i (pH 7.5) buffer with 5 mM DTT, and the solution was incubated at 37 °C for 10 min. After further incubation with 10 mM EDTA (pH 7.0) for 10 min and 15 mM MgSO 4 for another 10 min, the total membrane vesicles were harvested by centrifugation at 14,000 g for 25 min at 4 °C. The RSO vesicles were collected from the supernatant after centrifugation at 800 g for 12 min at 4 °C, then extensively washed and resuspended with 100 mM KP i (pH 7.5) at a protein concentration of ~20–28 mg ml −1 , frozen in liquid N 2 and stored at −80 °C. Melibiose transport assay with intact cells Melibiose active transport with intact cells were carried out with [1- 3 H]melibiose [4] , which was custom synthesized by PerkinElmer (Boston, MA). E. coli DW2 cells expressing MelB St were washed with 50 ml of 100 mM KP i (pH 7.5), so-called Na + -free buffer. The cell pellets were resuspended with 100 mM KP i (pH 7.5) and 10 mM MgSO 4 , adjusted to an A 420 =10 (~0.7 mg protein ml −1 ) and aliquoted with 50 μl. Transport was initiated by adding 2 μl of [ 3 H]melibiose with a specific activity of 10 mCi mmol −1 at a final concentration of 0.4 mM in the absence or presence of either 20 mM NaCl or LiCl, and stopped at a given incubation time. Intracellular melibiose was assayed by a fast filtration. Melibiose efflux and exchange assays RSO membrane vesicles containing the WT or a mutant MelB St in 100 mM KP i (pH 7.5) and 10 mM MgSO 4 were concentrated to ~28 mg ml −1 and pre-equilibrated overnight on ice with 20 mM [ 3 H]melibiose (10 mCi mmol −1 ), 0.75 μM monensin and 10 μM carbonylcyanide m-chlorophenylhydrazone [4] , [9] , [11] , without or with 20 mM NaCl or LiCl. Aliquots (2 μl) were diluted 200-fold into a given buffer in the absence (efflux) or presence (exchange) of 20 mM unlabelled melibiose [50] , and reactions were terminated by dilution and rapid filtration at a given time. Western blotting Twenty-five micrograms of RSO membranes were loaded onto each well of SDS–16% PAGE. After transfer onto the polyvinylidene difluoride membrane, MelB St proteins were detected with anti-His-tag antibody and imaged by the ImageQuant LAS 4000 Biomolecular Imager (GE Health Care Life Science) [47] . Trp→D 2 G FRET D 2 G (refs 4 , 9 , 43 , 47 , 59 ) was used to test affinity for the cosubstrate via FRET from Trp residues to the dansyl moiety of the D 2 G bound with MelB St . Steady-state fluorescence measurements were performed in a 3-mm quartz cuvette (Hitachi F-7000 Fluorescence Spectrophotomer or AMINCO-Bowman Series 2 Spectrometer). The purified sugar-free MelB St (1 μM) in the dialysis buffer or the buffer with 100 mM LiCl instead of NaCl was excited at wavelength of 290 nm and the emission fluorescence was recorded between 415 and 575 nm. With 10 μM D 2 G (the K D value for the WT [4] ), displacement of D 2 G bound by MelB St was carried out by adding 50 mM melibiose, methyl-β- D -thiogalactoside, glucose or sucrose, respectively. The difference spectra before and after the addition of a given sugar for displacement (Δ I ) is calculated and plotted. The RSO membrane vesicles prepared from DW2 cells expressing MelB St (1 mg ml −1 ) [4] , [9] in 100 mM KP i (pH 7.5) were excited at wavelength of 290 nm; the emission fluorescence at wavelength of 490 nm was recorded for 1 min after each of the following addition unless specified: (1) 10 μM D 2 G; (2) 20 mM NaCl or LiCl; (3) 50 mM NaCl or LiCl; (4) 120 mM melibiose or same volume of water. Half-maximal displacement of bound D 2 G (IC 50 ) Melibiose was added stepwise to the samples containing the RSO vesicles with D 2 G (10 μM) and 20 mM NaCl until no change in fluorescence emission occurred. The decrease in fluorescent intensity after each addition was corrected by the water dilution and was plotted as a function of melibiose concentration. The IC 50 value was determined by fitting a hyperbolic function to the data (OriginPro). Na + -stimulation constant ( K 0.5 ) for D 2 G FRET Applying the same experimental setup, NaCl was consecutively added to the sample containing the RSO vesicles and D 2 G (10 μM) [9] . An identical volume of water was used for the control. Fluorescent increase (Δ I , the difference before ( I 0 ) and after the addition of NaCl) was expressed as the percentage of the I 0 , corrected by a dilution effect, and then plotted as a function of Na + concentration. The K 0.5 for Na + simulation was determined by fitting a hyperbolic function to the data (OriginPro). Mutagenesis All MelB St mutants were constructed with the QuickChange Site-Directed Mutagenesis Kits (Stratagene) using the plasmid pK95 ΔAH/MelB St /CHis 10 as the template [4] . Gel filtration chromatography Gel filtration was performed in a Superdex 200 10/300 GL column on a Fast Protein Liquid Chromatography instrument. For the stability studies, the protein sample was placed at 23 °C for 5 days and analysed by the gel filtration chromatography and the D 2 G FRET assay. Precrystallization phospholipid treatment Before setting up crystallization trials, the protein samples were thawed out from −80 °C, ultracentrifuged at 384,492 g for 45 min at 4 °C (Beckman Coulter Optima MAX, TLA-100 rotor), diluted to a final protein concentration of 7 mg ml −1 and incubated with phospholipids at a concentration of 3.3 mM ( E. coli Extract Polar, Avanti, 100600) from a 15-mM stock dissolved with the dialysis buffer. Crystallization, data collection and processing Crystallization of MelB St was carried out by the hanging-drop vapour-diffusion method at 23 °C by mixing 2 μl of phospholipid-treated protein samples [60] containing 5 mM αNPG (4-nitrophenyl-α- D -galactopyranoside) with 2 μl reservoir containing 100 mM 2-(N-morpholino) ethanesulfonic acid (pH 6.5), 100 mM NaCl, 50 mM CaCl 2 , 35–37% PEG 400 and 0.08% octyl-β- D -galactopyranoside. Crystals were frozen with liquid nitrogen and tested for X-ray diffraction at the Lawrence Berkeley National Laboratory, ALS BL 8.2.1, 8.2.2, 5.0.1, 5.0.2 or at the Stanford Synchrotron Radiation Light Source BL 7-1 via remote data collection. The complete diffraction data set was collected at 100 K from a single cryocooled crystal at wavelength of 1.004 Å with an ADSC QUANTUM 315 detector at ALS BL 5.0.2; image data were processed with HKL 2000 (ref. 61 ) to a resolution of 3.35 Å with 98% completeness ( Table 1 ). Structure solution and refinement Data were processed in space groups P 3 2 21, P 3 1 21, P 3 2 and P 3 1 . The data set was analysed by Structure Factor Check on CCP4 (ref. 62 ) suite and Phenix Xtriage [63] , [64] , which indicated a strong off-origin peak at 0, 0, 0.5 along c* axis and also revealed merohedral twinning with twin fraction of 0.41 for the data processed in space groups P 3 2 and P 3 1 . Search probes were prepared using the server I-TASSER [65] , using the structures of MFS permeases, the inward LacY (PDB, 2V8N) and GlpT (1PW4), the occluded EmrD (2GFP), as well as the outward FucP (3O7Q). Using Phaser 2.52 programme [66] in Phenix suite, a single copy of each threading model with deletion of the longer loop 6–7 and loop 10–11 , and the C-terminal tail was used as the search probe to test the data processed in all space groups. Applying the native Patterson map and omit map to assist the molecular replacement processes, a maximal solution from the FucP-based MelB St model was identified, and the crystal symmetry was determined to be P 3 2 containing two additional pseudocrystallographic symmetries with 74% solvent content. The asymmetric unit contains four closely aligned molecules with two types of pseudo two-fold symmetry (twinning) along the b axis, with Mol-A and Mol-B related by 172°, and Mol-C and Mol-D related by 160° ( Supplementary Fig. S3 ). Mol-AB and Mol-CD are related by 0.5 pseudotranslation. Twin refinement was carried out by REFMAC 5.7 programme using the Jelly-Body-Restrained refinement option in CCP4 suite with the twinning operator k , h , - l . Initial refinement yielded R / R free of 0.37/0.42. Model verification was done by systematic calculation of omit maps at various regions. With iterative rounds of manual model building followed by simulated annealing and density modification, an interpretable density map to 3.35 Å resolution was obtained allowing assignment of most side chains for Mol-A and Mol-B ( Supplementary Figs S3c,d and S5a,b ). Final refinement was carried out using the Tangent Least-Square Jelly-Body-Restrained twin refinement, where the R / R free values dropped to 0.30/0.35 ( Table 1 ). As pseudosymmetries are present, higher apparent R / R free values are expected [67] . Out of 476 residues, 1–432 in Mol-A, regions 1–210 and 235–450 in Mol-B, 1–431 in Mol-C, as well as 1–100, 109–210, 235–398 and 408–431 in Mol-D, were well resolved. Residues (82.2%) are in most favoured, 17.4% in generously allowed and 0.4% in disallowed regions. Visualization of omit maps and manual model building were performed using Coot 0.7 (ref. 68 ). Surface electropotential maps were calculated using APBS software [69] . All crystallographic figures were generated with Pymol 1.5 (ref. 70 ). Accession codes: The protein coordinates and structure factor have been deposited in the Protein Data Bank with the accession number 4M64 . How to cite this article: Ethayathulla, A. S. et al . Structure-based mechanism for Na + /melibiose symport by MelB. Nat. Commun. 5:3009 doi: 10.1038/ncomms4009 (2014).